Photocurrent in graphene harnessed by tunable intrinsic plasmons Graphene’s optical properties in the infrared and terahertz can be tailored and enhanced by patterning graphene into periodic metamaterials with sub-wavelength feature sizes. Here we demonstrate polarization-sensitive and gate-tunable photodetection in graphene nanoribbon arrays. The long-lived hybrid plasmon–phonon modes utilized are coupled excitations of electron density oscillations and substrate (SiO 2 ) surface polar phonons. Their excitation by s-polarization leads to an in-resonance photocurrent, an order of magnitude larger than the photocurrent observed for p-polarization, which excites electron–hole pairs. The plasmonic detectors exhibit photo-induced temperature increases up to four times as large as comparable two-dimensional graphene detectors. Moreover, the photocurrent sign becomes polarization sensitive in the narrowest nanoribbon arrays owing to differences in decay channels for photoexcited hybrid plasmon–phonons and electrons. Our work provides a path to light-sensitive and frequency-selective photodetectors based on graphene’s plasmonic excitations. Graphene photodetectors rely on graphene for the absorption of light as well as the generation of an electrical signal through photovoltaic [1] , [2] , [3] , [4] , [5] , thermoelectric [6] , [7] , [8] , [9] or bolometric [10] , [11] , [12] mechanisms. However, the limited absorption in a single layer of graphene through inter-band transitions presents a key challenge [13] . Efforts to increase absorption include building microcavities around graphene [14] , [15] or enhancing the interaction with light through fabrication of quantum dots [16] , bowtie antennas [17] and other plasmonic nanostructures on top of the graphene [18] , [19] , [20] . Utilizing the Drude response of free electrons in combination with heavy chemical doping, an increased absorption reaching 40% in a single graphene layer has been achieved in the far-infrared [21] . Graphene with a moderate doping is usually very transparent in the mid-infrared wavelength range. However, the excitation of intrinsic graphene plasmons allows the tuning of strong absorption into the mid-infrared [22] , [23] , [24] . Intrinsic graphene plasmons also produce high confinement of electromagnetic energy in sub-wavelength dimensions in combination with a longer lifetime of the excitation as compared with plasmons in metals [25] . Moreover, unlike surface plasmons in metals [18] , [19] , [20] , [26] , plasmons in graphene can be effectively tuned with a backgate voltage, potentially enabling optoelectronic switching devices. In order to excite graphene plasmons with electromagnetic radiation, the wave vector and energy of plasmon and optical fields have to be matched, which can be done by light scattering from nearby nanostructures [27] , coupling by a grating fabricated on top or below the graphene [28] , or by patterning the graphene into periodic plasmonic metamaterials [29] , [30] , [31] . The latter approach is both simple and flexible in light of modern micro- and nano-fabrication techniques that allow sculpting graphene into a multitude of graphene superstructures. Arrays of graphene nanoribbons (GNRs), nanodiscs or nanorings can all support standing plasmons and can act as sharp notch filters in the mid-infrared, while staying more than 97% transparent elsewhere [29] , [30] , [31] . The dimensions, doping and, to a lesser degree, spacing between graphene nanostructures determine the position of the plasmon resonance and thus the absorption peak. Here, we incorporate arrays of GNRs, supporting standing plasmon excitations, as the active elements in graphene photodetectors. The graphene plasmons interact with surface polar (SP) phonons of the SiO 2 substrate forming long-lived hybrid plasmon–phonon modes with narrow spectral widths that allow efficient tuning of the mode by simple application of a gate voltage. The plasmon–phonon mode is excited in the mid-infrared exclusively under s-polarization, and upon its decay, electron and phonon temperatures in graphene are raised. The elevated temperatures can then result in changes in the electrical conductivity and thus a photocurrent. We distinguish between the effects of the phonon temperature ( T ph ) on the one hand and the electron temperature ( T e ) on the other: an increase in T ph leads to increased carrier-phonon scattering and a reduction in transport current (reduction mode), while an increase in T e is equivalent to an increased carrier density and leads to an increase in transport current (enhancement mode). Despite being a first demonstration of the intrinsic plasmonic-optoelectronic response in graphene metamaterials, our plasmon enhancement of the photoresponse reaches an order of magnitude under ambient conditions. We emphasize that the physical mechanism of enhancement reported here is fundamentally different from those in previously demonstrated integrated graphene photodetectors with metallic plasmonic structures [16] , [18] , [19] , [20] . Here, intrinsic graphene plasmonic properties are utilized, allowing for widely tunable plasmon resonance and light detection in the mid-infrared, an important wavelength range for a variety of crucial security, imaging and sensing applications. Standing plasmons in graphene superstructures Our photodetectors consist of GNR arrays with GNR widths between 80 and 200 nm, allowing us to match the standing plasmon resonance of the GNR array to the mid-infrared wavelength provided by a CO 2 laser (10.6 μm wavelength or a frequency of 943 cm −1 ). GNR arrays also impart on the device strong polarization anisotropy, where light polarized perpendicular to the GNR axis (s-pol.) can excite the plasmon, whereas light polarized parallel to the GNR (p-pol.) cannot. This can be used to differentiate between the effects of plasmonic excitations (collective electron density oscillations) and electron–hole pairs (single-particle excitations). An scanning electron microscopy image, a schematic of the experimental setup, and a schematic of the excitation and decay channels are displayed in Fig. 1 . Please see the Methods section for the experimental details. 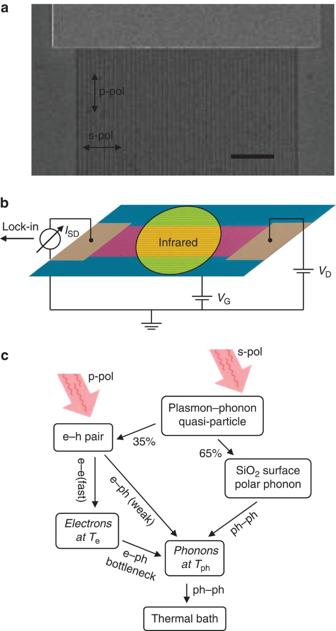Figure 1: GNR superlattice photodetector. (a) scanning electron microscopy close-up of the contact area of a GNR array photodetector with 100 nm GNR width and 100 nm GNR spacing. Scale bar, 2 μm. The length and width of the entire array are 30 and 10 μm, respectively. (b) Schematic of the photoconductivity setup. Infrared laser light at 10.6 μm is chopped at 1.1 KHz and the photocurrent is analysed by a lock-in amplifier referenced to the chopping frequency. (c) Illustration of the mechanism of phonon and hot electron generation through decay of the hybrid plasmon–phonon quasi-particles. S-polarized infrared light excites primarily the plasmon–phonon mode, while p-polarized light excites individual electron–hole pairs. The plasmon–phonon quasi-particle decays mainly through SP phonons into other phonons, while electron–hole pairs decay primarily into hot electrons. Electrons thermalize among themselves at a temperatureTe, and phonons among themselves at a temperatureTph. A bottleneck exists between electron and phonon baths, preventing full thermalization of electrons and phonons in graphene. This is especially important for the decay of electron–hole pairs excited with p-polarization. The type of scattering (electron–electron, electron–phonon or phonon–phonon) is indicated. Figure 1: GNR superlattice photodetector. ( a ) scanning electron microscopy close-up of the contact area of a GNR array photodetector with 100 nm GNR width and 100 nm GNR spacing. Scale bar, 2 μm. The length and width of the entire array are 30 and 10 μm, respectively. ( b ) Schematic of the photoconductivity setup. Infrared laser light at 10.6 μm is chopped at 1.1 KHz and the photocurrent is analysed by a lock-in amplifier referenced to the chopping frequency. ( c ) Illustration of the mechanism of phonon and hot electron generation through decay of the hybrid plasmon–phonon quasi-particles. S-polarized infrared light excites primarily the plasmon–phonon mode, while p-polarized light excites individual electron–hole pairs. The plasmon–phonon quasi-particle decays mainly through SP phonons into other phonons, while electron–hole pairs decay primarily into hot electrons. Electrons thermalize among themselves at a temperature T e , and phonons among themselves at a temperature T ph . A bottleneck exists between electron and phonon baths, preventing full thermalization of electrons and phonons in graphene. This is especially important for the decay of electron–hole pairs excited with p-polarization. The type of scattering (electron–electron, electron–phonon or phonon–phonon) is indicated. Full size image Plasmons are excited when the standing plasmon resonance of the graphene array, tuned by gate modulation of the chemical potential, coincides with a selected incident light frequency. These plasmons decay into hot electron–hole pairs via scattering from the edges of the nanostructures or via inelastic scattering with optical phonons [25] , [31] . Longer-lived hybrid plasmon–phonon modes that also have narrower spectral widths owing to the uncertainty principle can be induced through coupling with the underlying SiO 2 substrate [31] , [32] . SiO 2 supports SP phonons that are associated with a temporally changing electric field due to the vibrating positively and negatively charged atoms. On the surface of SiO 2 , this field penetrates outside and thus the SPs can couple to electronic excitations in neighbouring materials [32] , [33] , [34] . Graphene is the ultimately thin material and the SP coupling is particularly strong. Decay of hybrid plasmon–phonon modes leads to dissociation into hot electron–hole pairs and substrate SP phonons, which ultimately produce elevated electron and phonon temperatures ( Fig. 1c ). Direct decay into graphene optical phonons is precluded under our conditions, as the plasmon–phonon mode that we employ is situated below the optical phonon energy of graphene. Note that the decay channels of hybrid plasmon–phonon quasiparticles and electron–hole pairs are different, which together with the bottleneck for equilibration of electron and phonon temperatures opens up an avenue to control the temperatures of electrons and phonons by polarization. Dispersion and doping dependence of hybrid plasmon–phonons In freestanding graphene or graphene supported by nonpolar surfaces, such as diamond-like carbon, the plasmon resonance frequency follows a simple dispersion in the long wavelength limit, with q being the plasmon wave vector [22] , [35] , [36] . On the other hand, when graphene is placed on a polar substrate, such as SiO 2 or hexagonal boron nitride, the surface optical phonons can interact with the electronic degrees of freedom in graphene as described above, leading to coupled plasmon–phonon modes. Hybridization of plasmon and phonon modes alters their character, dispersion and lifetime [37] , [38] , [39] , [40] , [41] . 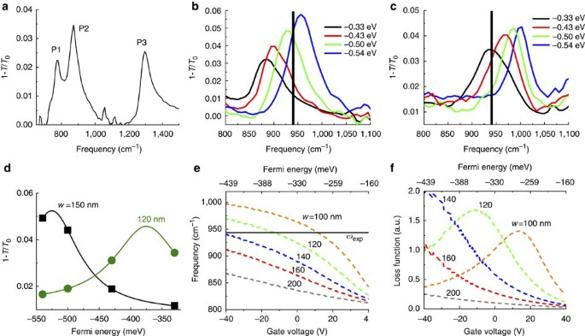Figure 2: Hybrid plasmon–phonon modes generated through coupling of graphene plasmons and SiO2SP phonons. (a) Extinction spectrum of a 160 nm GNR array on SiO2in the mid-infrared, measured with an Fourier transform infrared spectrometer under s-polarization (polarization perpendicular to the GNRs). Three hybrid plasmon–phonon modes can be identified. Their energies are determined by the interaction of the graphene plasmon mode with two SP phonons of the SiO2underlayer. (b,c) Extinction spectra in the region of the second peak (P2) for GNR arrays with GNR widths of (b) 150 nm and (c) 120 nm and varying chemical doping (Fermi) levels as indicated. The solid vertical line indicates the energy of the CO2laser used in subsequent photocurrent experiments. (d) Extinction as a function of doping, extracted from the two previous plots at the energy of the CO2laser, 943 cm−1. Black squares: 150 nm GNRs; green circles: 120 nm GNRs. The solid lines are Lorentzian fits. (e) Calculated plasmon resonance frequency as a function of Fermi energy and gate-voltage tuning for GNR arrays of different widths. (f) Calculated plasmon loss function as a function of Fermi energy and gate-voltage tuning for GNR arrays of different widths at the experimental frequency of 943 cm−1. Figure 2a shows an extinction spectrum measured on a GNR superlattice with 160-nm-wide GNRs. The extinction is defined in terms of the transmission through the array, measured with respect to similar wafers without graphene. Indeed, the extinction spectrum reveals resonances corresponding to the enhanced light absorption due to the excitation of hybrid plasmon–phonon modes that are only observed for polarization perpendicular to the GNRs (s-polarization). Three distinct resonances are observed owing to coupling of the graphene plasmon with two prominent SP phonons of SiO 2 over the frequency range of interest. Figure 2: Hybrid plasmon–phonon modes generated through coupling of graphene plasmons and SiO 2 SP phonons. ( a ) Extinction spectrum of a 160 nm GNR array on SiO 2 in the mid-infrared, measured with an Fourier transform infrared spectrometer under s-polarization (polarization perpendicular to the GNRs). Three hybrid plasmon–phonon modes can be identified. Their energies are determined by the interaction of the graphene plasmon mode with two SP phonons of the SiO 2 underlayer. ( b , c ) Extinction spectra in the region of the second peak (P2) for GNR arrays with GNR widths of ( b ) 150 nm and ( c ) 120 nm and varying chemical doping (Fermi) levels as indicated. The solid vertical line indicates the energy of the CO 2 laser used in subsequent photocurrent experiments. ( d ) Extinction as a function of doping, extracted from the two previous plots at the energy of the CO 2 laser, 943 cm −1 . Black squares: 150 nm GNRs; green circles: 120 nm GNRs. The solid lines are Lorentzian fits. ( e ) Calculated plasmon resonance frequency as a function of Fermi energy and gate-voltage tuning for GNR arrays of different widths. ( f ) Calculated plasmon loss function as a function of Fermi energy and gate-voltage tuning for GNR arrays of different widths at the experimental frequency of 943 cm −1 . Full size image In previous work [31] , we have studied extensively the dispersion of these hybrid plasmon–phonon modes and their associated damping processes in comparison with standard theory based on the random phase approximation. 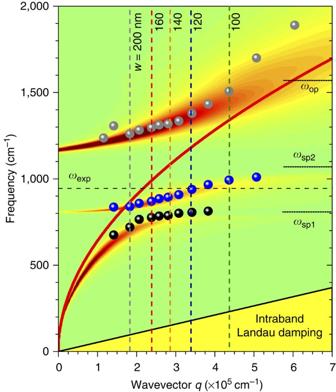Figure 3: Graphene’s loss function and plasmons. Colour intensity plot of graphene loss functionL(q,ω) assuming a doping of 0.33 eV. The calculation includes coupling with the intrinsic optical phonon and the two substrate polar phonons of SiO2as indicated in the figure. Prominent plasmon damping processes are included in the calculation with models taken from ref.30. SeeSupplementary Note 1for details of calculations. Data points are from absorption experiments such as inFig. 2a. Figure 3 plots the calculated random phase approximation plasmon loss function L ( q , ω ) in two-dimensional (2D) graphene, with details of the models and calculations documented in Supplementary Note 1 . Resonance positions of the coupled plasmon–phonon modes are extracted from the measured extinction spectra (symbols). The loss function describes both the plasmon–phonon mode dispersion and their resonance linewidth very well as detailed in ref. 31 . By slicing the graphene into a superlattice of GNRs each with a physical width of w , standing plasmons with momentum q = π /( w — w 0 ) are selected for. The denominator w — w 0 can be interpreted as the electronic width of the GNR, where w 0 is an experimentally determined fitting parameter [31] . Figure 3: Graphene’s loss function and plasmons. Colour intensity plot of graphene loss function L ( q , ω ) assuming a doping of 0.33 eV. The calculation includes coupling with the intrinsic optical phonon and the two substrate polar phonons of SiO 2 as indicated in the figure. Prominent plasmon damping processes are included in the calculation with models taken from ref. 30 . See Supplementary Note 1 for details of calculations. Data points are from absorption experiments such as in Fig. 2a . Full size image Plasmon–phonon modes are surface electromagnetic waves due to coupled excitations involving both collective electronic (plasmon) and ionic lattice oscillations (phonon). Analogous to a classical coupled harmonic oscillator problem, the nature and quality of the coupled mode (that is, phonon- or plasmon-like) depends on its resonant frequency. For example, a coupled mode resonating at frequency close to that of the SiO 2 SP phonon would exhibit narrow spectral width, inherited from the relatively long sub-picoseconds phonon lifetime [30] . Under certain physical situations, it is necessary to estimate the relative electromagnetic energy content distributed between the plasmon and phonon ‘oscillators’. For example, electron scattering with coupled plasmon–phonon mode [32] requires the knowledge of plasmon and phonon content as only the latter amounts to electron’s momentum relaxation. Here, we are interested in the plasmonic energy flow into the electronic and phononic baths, which drives the optoelectronic response in graphene. Over the range of energies E sampled in our experiments, we estimated the constituent electromagnetic energy content to be ~30–40% plasmon and ~60–70% phonon contents ( Supplementary Fig. S1 ). The plasmon–phonon mode whose frequency resides within the frequencies of the two SiO 2 SP phonons is shifted by chemical doping within the interval given by the two SP phonons ω sp1 and ω sp2 ( ∼ 800–1,100 cm −1 ) ( Fig. 2b ). We plot the resonance frequency position of this mode as a function of gate-voltage tuning for devices with different ribbon width in Fig. 2e . Our gate coupling allows for modulation of the Fermi energy within a 300 meV window. In conjunction with the sub-picoseconds lifetime of this hybrid plasmon–phonon mode, which translates to a broadening of ~100 meV, this should allow for gate-controlled switching of the plasmonic effect. At a photoexcitation frequency of ~943 cm −1 as indicated, our extinction measurements ( Fig. 2d ) and calculation ( Fig. 2f ) indeed suggest sufficient modulation of the plasmon loss function via gate-voltage tuning for GNR superlattices with GNR width of 140 nm and below. Plasmon-enhanced photoresponse Let us now first inspect the photoresponse of GNR superlattices with a fixed nanoribbon width of 140 nm. These superlattices display a large plasmonic photocurrent at a gate voltage near V G =−35 V as can be seen in Fig. 4a . Coupling of photons to the hybrid plasmon–phonon quasi particle is revealed by the order of magnitude increase in photocurrent for s-polarization (polarization perpendicular to the GNRs axis), and the strongly peaked gate-voltage characteristic of the photocurrent, in good agreement with the loss function for 140-nm GNR superlattices calculated in Fig. 2f . The plasmonic photocurrent has a full width at half maximum of ~40 V in gate voltage, which translate to ~100 meV in energy. This energy window can be made even smaller through improvements in electron mobility. Infrared light with p-polarization does not excite the standing plasmon, and the resulting weak photocurrent is owing to the excitation and subsequent decay of electron–hole pairs. Note that the photocurrent has negative sign throughout the gate-voltage range. This reduction mode photoconductivity is dominated by increased carrier scattering with photo-induced phonon temperature [12] . A spatial map of the plasmon-enhanced photoresponse is shown in the inset. The 30 μm × 10 μm GNR superlattice cannot be spatially resolved, because of the long wavelength of the CO 2 -laser photons, limiting our resolution to about 20 μm. 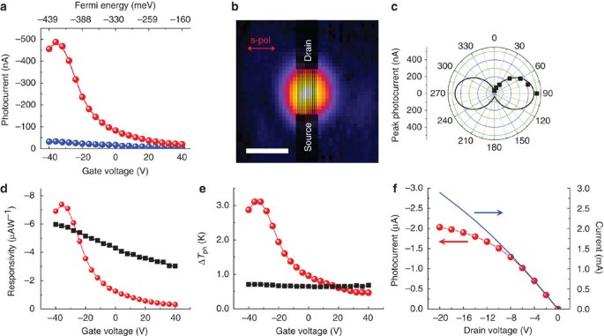Figure 4: Plasmon-enhanced graphene superlattice photodetector. (a) Gate-voltage-dependent photocurrent of a superlattice of 140 nm GNRs with incident infrared light under s-polarization (red spheres) and p-polarization (blue spheres). The corresponding Fermi energies are indicated on top. (Laser powerP=66 mW; drain voltageVD=−2 V.) (b) Scanning photocurrent image of the GNR superlattice photodetector. Scale bar, 30 μm. (c) Polarization dependence of the peak photocurrent under the same conditions. (d) Responsivity of 140 nm GNR superlattice (red spheres) and 2D graphene (black squares) upon photoexcitation with the same laser powerP=66 mW and drain voltageVD=−2 V. (e) Comparison of the lattice temperature increase of 140 nm GNR arrays (red spheres) and 2D graphene (black squares) under these conditions. (f) Bias dependence of the photocurrent and transport current in a 140 nm GNR superlattice atVG=−40 V. Photocurrent saturation sets in aboveVD=−8 V. Figure 4c plots the polarization angle dependence of the photocurrent, which follows a standard sine-square behaviour: Figure 4: Plasmon-enhanced graphene superlattice photodetector. ( a ) Gate-voltage-dependent photocurrent of a superlattice of 140 nm GNRs with incident infrared light under s-polarization (red spheres) and p-polarization (blue spheres). The corresponding Fermi energies are indicated on top. (Laser power P =66 mW; drain voltage V D =−2 V.) ( b ) Scanning photocurrent image of the GNR superlattice photodetector. Scale bar, 30 μm. ( c ) Polarization dependence of the peak photocurrent under the same conditions. ( d ) Responsivity of 140 nm GNR superlattice (red spheres) and 2D graphene (black squares) upon photoexcitation with the same laser power P =66 mW and drain voltage V D =−2 V. ( e ) Comparison of the lattice temperature increase of 140 nm GNR arrays (red spheres) and 2D graphene (black squares) under these conditions. ( f ) Bias dependence of the photocurrent and transport current in a 140 nm GNR superlattice at V G =−40 V. Photocurrent saturation sets in above V D =−8 V. Full size image Here, I Plasmon and I e−h are the photocurrents due to the plasmon–phonon mode and electron–hole pairs, respectively, and φ is the polarization angle, defined as φ =0° for p-polarization. Enhanced light absorption due to localized plasmons and their subsequent decay primarily into phonons is responsible for the observed enhancement factor β =| I 90° / I 0° | on the order of ~15, to be discussed. A comparison between the photoresponse of a GNR superlattice and 2D graphene of the same overall dimension (30 μm × 10 μm) is shown in Fig. 4d . The peak responsivity of the 140 nm GNR superlattice is slightly larger than that of 2D graphene. Note that this quantity can easily be increased in both cases by increasing the drain voltage, making the device shorter or increasing the thermal resistance of the gate stack. By calibrating with the very different transport currents and plotting Δ G / G instead ( Supplementary Fig. S2 ), a six times larger response for the GNR superlattice is obtained. ( G is the conductance and Δ G=I ph / V D is the photoconductance.) We can go a step further and extract the lattice temperature increase upon photoexcitation by measuring the temperature dependence of the transport current in a cryostat around room temperature: Δ G /( G Δ T ph )=−3.1 × 10 −4 K −1 and Δ G /( G Δ T ph )=−2.5 × 10 −4 K −1 for 140 nm GNRs and 2D graphene, respectively. Here Δ T ph is the lattice temperature increase. The resulting curves are plotted in Fig. 4e . Within the plasmon–phonon resonance, the superlattice shows a lattice temperature increase of 3.1 K above room temperature, while the 2D graphene lattice temperature increase is flat at 0.7 K. Typical absorption for graphene superlattices on the order of 5% ( Fig. 2d ) and for 2D graphene in the Pauli blocking regime around 1% are consistent with these temperature increases inferred from the photocurrents. The drain-voltage dependence of the plasmon-enhanced photocurrent ( Fig. 4f ) shows saturation starting at 8 V of source-drain bias corresponding to 0.26 V μm −1 on average. The associated decrease in photoconductance Δ G ( Supplementary Fig. S3 ) is partly owing to the increased temperature stemming from Joule heating and partly owing to inhomogeneous broadening of the plasmon resonance due to the potential gradient along the graphene at higher drain voltages. To first order, the deposited electrical power P el =| V D I | is proportional to the increased device temperature relative to its ambient, denoted as Δ T Joule . A simple estimate based on our previous work suggests Δ T Joule / P el ~10 3 KW −1 for 30 μm × 10 μm large devices [42] . Source-drain voltages between 2 and 20 V correspond to deposited electrical powers between 1 and 60 mW, and temperature increases between 1 and 60 K. We can identify two contributions to the decrease in photoconductance with Joule heating, both discussed in more detail in the Supplementary Fig. S3 . First, Joule heating leads to an increase in the out-of-plane thermal conductance of graphene due to the SiO 2 /Si gate stack κ 0 , which reduces the photo-induced lattice temperature increase Δ T ph through Δ T ph = P ph / κ 0 , where P ph is the absorbed power by the phonon bath. Second, Joule heating also leads to a broadening of the gate-voltage-tuned plasmonic photocurrent peak owing to a reduction in plasmon lifetime. This effect is small, however, less than 10% for 10 V source-drain bias. Dual tunability of plasmonic graphene photodetectors We now turn to the GNR width dependence of the plasmon-enhanced photocurrent, which lets us tune the peak photoresponse in addition to gate-voltage tuning. 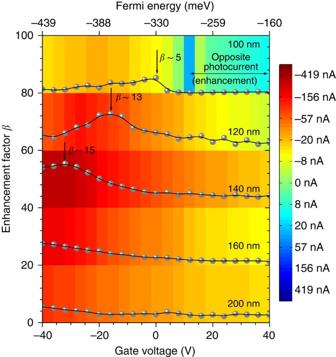Figure 5: Photoresponse as a function of gate-voltage tuning and GNR width. Gate-voltage-dependent photocurrent enhancement factorβ=|I90°/I0°| for GNR superlattices with different GNR width. Subsequent curves are displaced by 20 units for clarity. Photocurrent enhancement owing to the plasmon reachesβ=15 for 140-nm GNR superlattices. Colour coding: gate-voltage-dependent photocurrentIphfor these GNR superlattices under s-polarization (I90°), plotted on a logarithmic colour scale. (P=66 mW,VD=−2 V). The entire data set for s- and p-polarization is shown inFig. 6. Figure 5 plots the experimental photocurrent under polarization normal to the GNR axis, as well as the photocurrent enhancement factor β =| I 90° / I 0° | for GNR superlattices of different widths. The photocurrent enhancement factors can be compared with the modelled absorption peaks in Fig. 2f . Both the 140 and 120 nm photocurrent peaks match very well with the corresponding maxima in the loss function. In 200 and 160-nm GNRs, the photocurrent peak resides outside our experimental range of V G =−40 to 40 V in both theory and experiment. For the smallest GNRs with width of 100 nm and below, however, the photocurrent peak is weaker and shifted as compared with the modelled absorption peak. Interestingly, we also observe inversion of the photocurrent direction in 100 and 80-nm GNR arrays at positive gate voltages, and a distinct photocurrent polarity dependence on the polarization of the incident light at certain gate voltages as indicated by the brown-shaded regions in Fig. 6 . We proceed to discuss the photocurrent generation mechanisms in order to explain these observations. Figure 5: Photoresponse as a function of gate-voltage tuning and GNR width. Gate-voltage-dependent photocurrent enhancement factor β =| I 90° / I 0° | for GNR superlattices with different GNR width. Subsequent curves are displaced by 20 units for clarity. Photocurrent enhancement owing to the plasmon reaches β =15 for 140-nm GNR superlattices. Colour coding: gate-voltage-dependent photocurrent I ph for these GNR superlattices under s-polarization ( I 90° ), plotted on a logarithmic colour scale. ( P =66 mW, V D =−2 V). The entire data set for s- and p-polarization is shown in Fig. 6 . 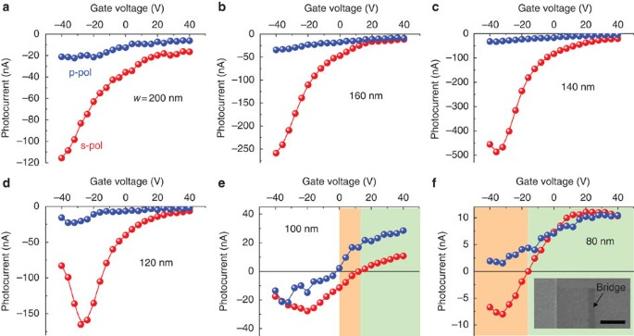Figure 6: Photocurrent polarity for varying GNR width. (a–f) Photocurrent under s- and p-polarization as a function of gate-voltage tuning for arrays with varying GNR width. (P=66 mW,VD=−2 V). For p-polarized light, which does not excite the plasmons, the photocurrent is more negative at negative gate voltages, owing to the stronger reduction mode photocurrent at higher electrostatic doping12. S-polarized light excites the plasmon–phonon mode and the photocurrents are dominated by the plasmonic response. GNR arrays above 120 nm width (a–d) show reduction mode photoconductivity throughout the gate-voltage range. The smallest GNRs (100 and 80 nm, (e–f)) exhibit transitions from negative to positive photocurrent with increasing gate voltage owing to a switch from reduction mode to enhancement mode photoconductivity. The green-shaded gate-voltage regions indicate positive photocurrent. The brown-shaded regions highlight the gate-voltage ranges where s- and p-polarization yield oppositesignof photocurrent. The 80-nm GNR array contains seven graphene bridges perpendicular to the GNRs to guarantee current continuity along the 30-μm-long GNR array. One of the bridges is shown in the zoomed-in scanning electron microscopy image in the inset in (f). Scale bar, 2 μm. Full size image Figure 6: Photocurrent polarity for varying GNR width. ( a – f ) Photocurrent under s- and p-polarization as a function of gate-voltage tuning for arrays with varying GNR width. ( P =66 mW, V D =−2 V). For p-polarized light, which does not excite the plasmons, the photocurrent is more negative at negative gate voltages, owing to the stronger reduction mode photocurrent at higher electrostatic doping [12] . S-polarized light excites the plasmon–phonon mode and the photocurrents are dominated by the plasmonic response. GNR arrays above 120 nm width ( a – d ) show reduction mode photoconductivity throughout the gate-voltage range. The smallest GNRs (100 and 80 nm, ( e – f )) exhibit transitions from negative to positive photocurrent with increasing gate voltage owing to a switch from reduction mode to enhancement mode photoconductivity. The green-shaded gate-voltage regions indicate positive photocurrent. The brown-shaded regions highlight the gate-voltage ranges where s- and p-polarization yield opposite sign of photocurrent. The 80-nm GNR array contains seven graphene bridges perpendicular to the GNRs to guarantee current continuity along the 30-μm-long GNR array. One of the bridges is shown in the zoomed-in scanning electron microscopy image in the inset in ( f ). Scale bar, 2 μm. Full size image Biased photodetectors either work in a mode where the transport current is enhanced or reduced owing to the absorbed energy. Enhancement, prominent in semiconductor bolometers including gapped bilayer graphene [11] , is promoted by the conduction of the photo-generated carriers and can be described in graphene by a hot electron temperature T e (refs 8 , 9 ), while reduction is mediated through the phonon-limited mobility, and thus can be described by the raised lattice temperature T ph . Enhancement dominates in graphene at low doping close to the Dirac point, while reduction dominates at high doping [12] . As our GNR superlattices are strongly p-doped, with an estimated Dirac point at V G =52 V, reduction due to increased phonon scattering usually dominates. Indeed, 120, 140, 160 and 200-nm-wide GNR superlattices show the reduction mode throughout the gate voltage range from −40 V to 40 V, and Fig. 4c plots the corresponding lattice temperature increase Δ T ph in the case of the 140-nm GNR superlattice. In narrower GNRs with widths around 100 nm and below, however, the situation is different. Here, disordered edges lead to a thermally activated hopping transport along localized states with size close to the GNR width [43] . The resulting transport gap (or mobility gap) on the order of 100 meV is not to be confused with a real bandgap, which becomes important only for much narrower GNRs below 10 nm (ref. 44 ), or in bilayer graphene [11] , where the bandgap is even tunable by a perpendicular electric field. In GNRs, the energy scale of the transport gap derives from both localization and charging, and translates into a gate-voltage window of a few volts around the Dirac point. The activation energy for hopping transport within the transport gap is on the order of 10 meV (ref. 43 ), suggesting that an increase in electron temperature upon photoexcitation should lead to a positive photocurrent when biased in the vicinity of the mobility gap gate-voltage region. Thus, we would expect that we see a transition from reduction mode to enhancement mode in small-width GNRs, and that this transition moves to more negative gate voltages for narrower GNRs. In our experiments, we indeed observe a positive photocurrent in 100-nm-wide GNR arrays above V G =10 V, and in 80-nm-wide GNR arrays above V G =−20 V ( Figs 5 and 6 ). An interesting situation occurs when the position of the plasmonic absorption peak, which moves to more positive gate voltages as the nanoribbon width is reduced, crosses over from reduction mode to enhancement mode. In 100-nm-wide GNR arrays, the plasmonic absorption peak ( Fig. 2f ) lies in a region of reduced photosensitivity owing to the competition between reduction mode and enhancement mode photoconducitvity. This certainly contributes to the comparatively small enhancement factor β ~5 in 100 nm GNRs, in combination with a broadening of the plasmon peak owing to edge scattering [31] . In 80-nm-wide GNR arrays ( Fig. 6f ), the plasmon peak has become very broad owing to edge scattering, so that plasmon enhancement extends over a wide gate-voltage range in both reduction mode and enhancement mode regions. It is in these narrowest of our GNRs where we observe a switch in photocurrent sign as a function of incident light polarization in addition to gate voltage. P-polarized light excites electron–hole pairs, which decay through electron–electron scattering, effectively multiplying the primary photocarriers, and leading to an enhancement-mode photocurrent owing to the increased electron temperature (see also the schematic in Fig. 1c ). Thermalization with phonons is hindered through an electron–phonon scattering bottleneck [8] , [9] . S-polarized light, on the other hand, excites the hybrid plasmon–phonon mode, which decays mainly into phonons owing to the 65% phonon character of this mode. This increases electron–phonon scattering (reduction mode) and leads to a photocurrent in the opposite direction. The photocurrent sign, not only the magnitude, therefore depends on the polarization of the incident light within a gate-voltage range where enhancement and reduction mode photoconductivity are of the same order. As far as we know, the photocurrent polarity change with polarization has not been reported in any other material system before. It is a consequence of the competition between enhancement mode, which is favoured by the decay of electron–hole pairs, and reduction mode, which is favoured by the decay of the hybrid plasmon–phonon quasiparticles. In conclusion, we present a novel room-temperature mid-infrared detector based on the intrinsic graphene plasmon excitations. Graphene plasmons are longer lived than their counterparts in metals because of the superior mobility in graphene. We further alter the graphene plasmons by remote plasmon–phonon coupling with the surface phonons of the polar substrate. The hybrid plasmon–phonon modes are even longer lived and highly gate tunable. We obtain very promising plasmonic enhancement factors with GNR superlattice photodetectors, exceeding an order of magnitude as compared with excitation of electron–hole pairs alone. The general principle can be applied to engineering graphene photodetectors for applications over very wide spectra from terahertz to infrared frequencies. Future improvements include low-temperature operation, device geometry optimizations, interdigitated finger electrodes, access to the higher-energy plasmon–phonon mode whose wavefunction has higher plasmon character and more effective grating structures instead of nanoribbons that preserve graphene’s intrinsic high mobility. Sample preparation Single-layer graphene ( Supplementary Fig. S4 ) is grown by CVD on copper foil [45] . The copper is dissolved in etchant CE200 and the free-floating graphene is transferred to a silicon chip with 90 nm SiO 2 . Graphene devices 30 μm long and 10 μm wide, as well as the 1/20/40 nm Ti/Pd/Au contacts are fabricated by e-beam lithography. In a final step, the 2D graphene is etched into GNR superlattices by e-beam lithography with PMMA resist and oxygen plasma. The nanoribbon widths range from 80 to 200 nm. The fill factor (width/period=1/2) is kept constant throughout. Experimental details GNR superlattice photodetectors are illuminated by a focused and chopped CO 2 -laser beam at λ =10.6 μm or ω =943 cm −1 . We use a ZnSe objective to focus the laser to a spot 20 μm in diameter. The laser power is 66 mW, corresponding to a moderate power density on the order of 2 × 10 4 W cm −2 . In plasmon-enhanced photodetectors, the typical p–n junction geometry would be undesirable, as junctions include doping gradients that lead to shifts in plasmon frequencies, broadening the phonon–plasmon peaks. Therefore, we chose to apply a small drain bias of −2 V (corresponding to an average electric field of 670 V cm −1 ) keeping the electrostatic doping almost constant throughout. The source side is connected to a preamplifier and lock-in detector, referenced to the chopping frequency of the mechanical chopper at 1.1 KHz ( Fig. 1c ). The root mean square values of the photocurrent amplitude at the lock-in output are translated to peak-to-peak values for the manuscript. Measurements are performed in air, and the electrical characteristic of the GNR superlattice photodetectors are p-type ( Supplementary Fig. S5 ) with residual doping corresponding to a Fermi level of E F =0.33 eV. A global Si backgate is used to tune the Fermi level. How to cite this article: Freitag, M. et al . Photocurrent in graphene harnessed by tunable intrinsic plasmons. Nat. Commun. 4:1951 doi: 10.1038/ncomms2951 (2013).